TERRA transcripts are bound by a complex array of RNA-binding proteins Telomeres are specialized heterochromatin structures at the ends of eukaryotic chromosomes that prevent chromosome ends from being recognized as DNA double-strand breaks [1] , [2] . In vertebrates, telomeres are composed of TTAGGG repeats bound by a six-protein complex known as shelterin [3] , [4] . Despite the long-standing belief that telomeres were transcriptionally inactive because of their compact heterochromatin structure, two independent reports recently showed that telomeres are transcribed [5] , [6] . In particular, the telomeric C-rich strand is transcribed by the DNA-dependent RNA polymerase II, giving rise to UUAGGG-repeat transcripts known as TERRA/TelRNAs (referred hereafter as TERRA) [5] , [6] . TERRA are non-coding RNAs, heterogeneous in size (ranging between 100 bp and 9 kb) and formed by a combination of subtelomeric and telomeric sequences [5] , [6] . To date, transcripts containing telomeric repeats have been described in Mus musculus , Homo sapiens , Saccharomyces cerevisiae and Danio rerio [5] , [6] , [7] . TERRA have been detected at telomeres, as indicated by their co-localization with shelterin components such as TRF1 [5] , [6] , suggesting that TERRA are novel structural components of telomeres. TERRA levels are modulated by a number of factors, including telomeric chromatin status, cellular stresses, as well as during ontogenesis and cancer [6] . More recently, TERRA abundance was shown to be tightly regulated during nuclear reprogramming of differentiated cells into induced pluripotent stem cells, highlighting the importance of TERRA regulation during the acquisition of a pluripotent state (Marion et al [8] ; reviewed in Schoeftner and Blasco [9] ). Until recently, however, the trans -acting factors (for example, RNA-binding proteins (RBPs), miRNAs, and so on) and the mechanisms controlling TERRA levels remained unaddressed. A recent report described the shelterin protein TRF2 as a novel TERRA-interacting protein, thereby facilitating heterochromatin formation and recruitment of the replication–initiation ORC complex to telomeres [10] . Previous reports suggested that RBPs are important for telomere biology. In particular, members of the heterogeneous nuclear ribonucleoprotein family (hnRNPs), which participate in many aspects of mRNA maturation/turnover, have been proposed to regulate both telomere length and telomerase. Among these, hnRNP A1, A2B1, A3, D (also known as AUF1) and E can associate with the single-stranded telomeric repeats, and hnRNP A1 has been shown to influence telomere length [11] , [12] , [13] (reviewed in Ford et al . [14] ). In addition, hnRNP A1, D and C1/C2 were shown to interact with human telomerase [12] , [15] , [16] , [17] , [18] . The hnRNP proteins can also affect chromatin remodelling and transcription in a DNA-independent manner through protein–protein interactions (for example, hnRNP U binds RNA polymerase II) (reviewed in Carpenter et al . [19] ). The hnRNP A1 and D have been also implicated in transcription owing to their ability to bind to and unwind G-quadruplexes [18] , [20] . A role for hnRNP A1 in transcription that does not involve unwinding of G-quadruplexes has been also reported [21] . Another group of RBPs, known to bind to small nucleolar RNAs, including GAR1 and dyskerin, has also been found to interact and regulate telomerase in vivo [22] , [23] . Here, we report the identification of the RBPs bound to TERRA in primary mouse embryonic fibroblasts (MEFs). We found that hnRNPs are the RBPs that bind more abundantly to TERRA. Furthermore, we show that these RBPs regulate TERRA abundance as well as TERRA location to telomeres. Moreover, downregulation of TERRA-bound RBPs can impact on telomere length and DNA damage at telomeres. Identification of TERRA-bound RBPs in primary MEFs Here, we carried out an unbiased analysis searching for the specific set of RBPs that bind to mouse TERRA. To identify the TERRA-bound RBPs, we performed biotin pull-down assays using a biotinylated transcript consisting of eight UUAGGG repeats (8×UUAGGG) and nuclear extracts from primary MEFs. Two mass spectrometry (MS) approaches were used for the identification of RBPs after pull-down assays (1) liquid chromatography–matrix-assisted laser desorption/ionisation–tandem MS (LC-MALDI-MS/MS) analysis of pull-down material and (2) matrix-assisted laser desorption/ionisation–time of flight/time of flight–MS (MALDI TOF/TOF-MS) analysis of excised bands obtained after SDS–polyacrylamide gel electrophoresis (SDS–PAGE) separation and Coomassie staining of pull-down material. A biotinylated control RNA corresponding to a random sequence of the same length as the biotinylated TERRA (N 48 ) was used for differential identification in both approaches. 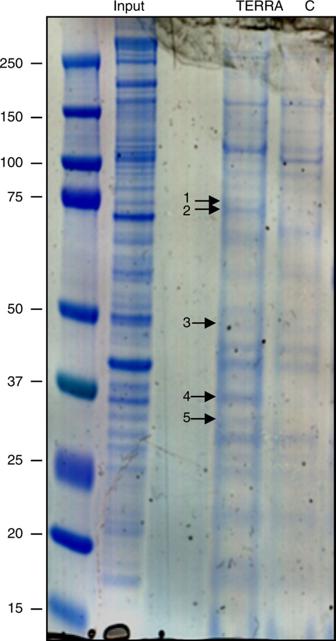Figure 1: Identification of the most abundant RBPs bound to TERRA. Biotin pull-down assays followed by SDS–PAGE separation were used to isolate TERRA-bound RBPs. Biotinylated TERRA transcripts were incubated with nuclear protein lysates from primary MEFs, whereupon RBPs were separated and detected by SDS–PAGE followed by Coomassie staining; excised bands were then subjected to LC-MALDI TOF/TOF-MS analysis. Band 1: hnRNP M, band 2: hnRNP M, band 3: hnRNP F, band 4: hnRNP A1 and hnRNP A2/B1 and band 5: hnRNP A2/B1. A biotinylated control RNA (C) corresponding to a random sequence of the same length as the biotinylated TERRA (N48) was used for differential identification. Input is the nuclear protein lysate. Molecular weight markers are shown in kDa. The first approach led to the identification of some 41 candidates that were bound only to the biotinylated TERRA and not to the control RNA ( Table 1 ). More than 50% of the identified candidates possess known RNA-binding domains ( Table 1 ) and locate predominantly in the nucleus. Interestingly, some of the identified RBPs have been previously reported to participate in regulation of telomeres and telomerase, as mentioned above. In particular, hnRNP A1, A2B1 and D/AUF1 bind to telomeres [11] , [12] , [13] (reviewed in Ford et al . [14] ) and hnRNP A1, D and GAR1 bind to telomerase [12] , [15] , [16] , [22] . The second approach allowed the identification of those RBPs that bind more abundantly to the biotinylated TERRA ( Fig. 1 ). Importantly, the proteins identified by this second approach were among those identified by the first approach, confirming the robustness of their interaction with TERRA. Virtually, all the RBPs identified by the second approach belonged to the hnRNP family, including hnRNP A1, A2/B1, M and F, by order of abundance ( Fig. 1 ). While in preparation of this manuscript, a different group independently found that hnRNP A1, A2/B1 and M bound to human TERRA transcripts [10] , although this interaction was not further characterized in the paper. Here, we set out to show the in vitro and in vivo binding of these proteins to TERRA and to study their role in TERRA regulation and telomere biology. Table 1 TERRA-bound proteins identified by LC-MALDI-MS/MS. Full size table Figure 1: Identification of the most abundant RBPs bound to TERRA. Biotin pull-down assays followed by SDS–PAGE separation were used to isolate TERRA-bound RBPs. Biotinylated TERRA transcripts were incubated with nuclear protein lysates from primary MEFs, whereupon RBPs were separated and detected by SDS–PAGE followed by Coomassie staining; excised bands were then subjected to LC-MALDI TOF/TOF-MS analysis. Band 1: hnRNP M, band 2: hnRNP M, band 3: hnRNP F, band 4: hnRNP A1 and hnRNP A2/B1 and band 5: hnRNP A2/B1. A biotinylated control RNA (C) corresponding to a random sequence of the same length as the biotinylated TERRA (N 48 ) was used for differential identification. Input is the nuclear protein lysate. Molecular weight markers are shown in kDa. Full size image The hnRNPs bind to TERRA in vitro and in vivo We first performed biotin pull-down assays followed by western blot using specific antibodies against hnRNP A1, A2B1, F and M to confirm our protein identification results ( Fig. 2a ). Because of the labile nature of TERRA (half-life of ∼ 3 h), we also tested for the presence of hnRNP D/AUF1 (which was identified by the first approach; Table 1 ) and of HuR in TERRA. Both hnRNP D/AUF1 and HuR belong to the AU-rich binding protein family, and are the best-studied RBPs implicated in controlling mRNA turnover (reviewed in Brennan and Steitz [24] , Barreau et al . [25] and Guhaniyogi and Brewer [26] ). 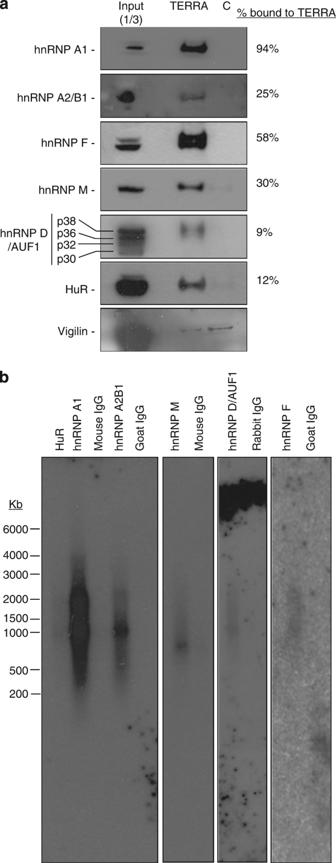Figure 2:In vitroandin vivovalidation of TERRA-bound RBPs identified by LC-MALDI TOF/TOF-MS analysis. (a) Biotinylated TERRA transcripts were incubated with nuclear protein lysates from primary MEFs and their association with hnRNP A1, A2B1, F, M, D/AUF1 and HuR was detected by western blotting. A biotinylated control RNA (C) corresponding to a random sequence of the same length as the biotinylated TERRA (N48) was used as control for specificity. The RBP vigilin was used to monitor the evenness of sample input, as it was identified in both TERRA and control samples by LC-MALDI. Quantification of the TERRA signal/input ratio was carried out to assess the amount of endogenous RBPs bound to TERRA (see % bound to TERRA). (b) Immunoprecipitation (IP) assay using 3 mg of nuclear extracts prepared from primary MEFs and 30 μg of either RBPs antibodies or IgG1, under conditions that preserved mRNP complexes. RNAs isolated from IP material were subjected to northern blotting and hybridized with a32P-dCTP-labelled 1.6 kb telomeric probe. Size markers are shown in Kb. As shown in Figure 2a , hnRNP A1, A2B1, F, M, D/AUF1 and HuR formed complexes only with the biotinylated TERRA and not with the control RNA. The RBP vigilin served to monitor the evenness of sample input, as it was identified in both 8×UUAGGG and control (N 48 ) samples by LC-MALDI ( Fig. 2a ). Quantification of the TERRA signal/input ratio signal showed that hnRNP A1 and hnRNP F are the RBPs more abundantly bound to TERRA ( Fig. 2a ). Figure 2: In vitro and in vivo validation of TERRA-bound RBPs identified by LC-MALDI TOF/TOF-MS analysis. ( a ) Biotinylated TERRA transcripts were incubated with nuclear protein lysates from primary MEFs and their association with hnRNP A1, A2B1, F, M, D/AUF1 and HuR was detected by western blotting. A biotinylated control RNA (C) corresponding to a random sequence of the same length as the biotinylated TERRA (N 48 ) was used as control for specificity. The RBP vigilin was used to monitor the evenness of sample input, as it was identified in both TERRA and control samples by LC-MALDI. Quantification of the TERRA signal/input ratio was carried out to assess the amount of endogenous RBPs bound to TERRA (see % bound to TERRA). ( b ) Immunoprecipitation (IP) assay using 3 mg of nuclear extracts prepared from primary MEFs and 30 μg of either RBPs antibodies or IgG1, under conditions that preserved mRNP complexes. RNAs isolated from IP material were subjected to northern blotting and hybridized with a 32 P-dCTP-labelled 1.6 kb telomeric probe. Size markers are shown in Kb. Full size image Next, we conducted in vivo binding assays to test association of the RBPs to endogenous TERRA. To this end, we isolated RNA from RBP-immunoprecipitated (IP) material ( Supplementary Fig. S1 ) followed by northern blot hybridization using a specific probe to detect TERRA transcripts. As shown in Figure 2b , TERRA signal was detected in HuR-, hnRNP A1-, A2B1-, M-, D- and F-IPs and not in control immunoglobulin G (IgG)-IP samples, showing the in vivo binding of these RBPs to TERRA. Collectively, these results indicate that TERRA are bound in vivo by a complex set of RBPs in which different members of the hnRNP family are the most abundant ones. TERRA-bound RBPs influence TERRA abundance and location To assess the functional consequences of RBP-TERRA interactions, we first measured TERRA levels after knocking down expression of RBPs. This was achieved by transient transfection of primary MEFs with specific small interfering RNAs (siRNAs) against the different RBPs identified here. We were able to knockdown RBPs proteins to ∼ 10–50% of the levels present in primary MEFs transfected with a control siRNA ( Fig. 3a ). We next measured TERRA levels by northern blot analysis using total RNA from siRNA-transfected MEFs ( Fig. 3b ). For all of the siRNAs against TERRA-interacting RBPs tested here, lowering of RBP expression by 10–50%, showed a tendency to increase TERRA steady-state levels compared with control-transfected cells, this difference was more dramatic in hnRNP F, M and D/AUF1 knockdowns and reached statistical significance in the case of hnRNP F knockdown ( Fig. 3b ; see also Supplementary Fig. S2a ). These results indicate that hnRNP F may act as a potent repressor of TERRA levels. This repression might be linked to the known role of hnRNP F as a negative regulator of pre-mRNA cleavage, which is needed for the polyadenylation steps [27] . In particular, hnRNP F downregulation may result in increased polyA+-TERRA contributing to augmented protection of 3′ end of TERRA from exonucleases, which in turn could increase TERRA stability and the observed increase in TERRA levels. We could not detect clear changes in the extent of polyadenylation after hnRNP F knockdown as compared to C siRNA ( Supplementary Fig. S2 ). However, the interpretation of these results should be taken with caution given the heterogeneity in TERRA size, as well as the fact that TERRA levels also change upon RBPs siRNAs ( Fig. 3b and Supplementary Fig. S2 ). For these reasons, we next focused on studying changes in mRNA stability. We determined TERRA half-life ( t 1/2 ) after treatment with actinomycin D, which inhibits de novo transcription. Interestingly, knockdown of hnRNP F increased the half-life of TERRA to an estimated t 1/2 > 8 h compared with t 1/2 =5.7 h in the control-transfected cells ( Fig. 3c ). Of interest, we observed a reproducible increase in TERRA levels at the 4-h time point of actinomycin D treatment, which could be associated to a transient stabilization of TERRA due to the translocation of stabilizing RBPs to the cytoplasm on actinomycin D treatment (for example, see HuR translocation in Supplementary Fig. S3a ). As a control for the former treatment, we measured the half-life of the labile c-fos mRNA by reverse transcriptase quantitative PCR in parallel with the half-life of a stable transcript, the GAPDH mRNA [28] . As expected, the c-fos mRNA decayed rapidly on actinomycin D incubation, with a half-life of 1.5 h, whereas GAPDH mRNA decayed at slower rates, with a half-life of 7 h ( Supplementary Fig. S3b ). Note that c-fos mRNA, a target of HuR [28] , also becomes stabilized at the 4-h time point. Interestingly, the TERRA half-life value falls in between the half-life of the labile mRNA, c-fos ( t 1/2 =1.51 h), and the stable mRNA, GAPDH ( t 1/2 =7.07 h) ( Supplementary Fig. S3b ). Different increases in TERRA stability were also observed on downregulation of the other TERRA-bound RBPs ( Supplementary Fig. S4 ). As some of the hnRNPs are known to participate in the nuclear export of mRNAs [19] , [29] , we also tested the possibility of changes in the subcellular localization of TERRA on the siRNAs of RBPs. TERRA remained nuclear ( Supplementary Fig. S5 ), in agreement with their reported presence restricted to the nuclear compartment when TERRA were first described [5] , [6] . Collectively, these results suggest that hnRNP F represses TERRA levels, at least in part, by reducing the stability of TERRA transcripts and this effect is probably independent of TERRA polyadenylation status. 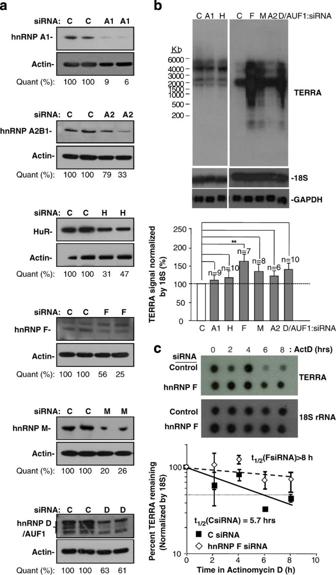Figure 3: TERRA-bound RBPs regulate TERRA levels. (a) At 2 days after siRNA transfection, primary MEFs were harvested for western blot analysis to monitor RBP expression; whole-cell extracts (20 μg) were used to detect hnRNP A1 (A1), HuR (H) and hnRNP D/AUF1 (D) and nuclear extracts (50 μg) to detect hnRNP A2B1 (A2), hnRNP F (F) and hnRNP M (M). Duplicates of each transfection are shown. β-Actin was used as loading control. Quantification of RBP protein levels (%) relative to control transfection (C) is indicated in the bottom of each panel. (b) Northern blotting using a32P-dCTP-labelled 1.6 kb telomeric probe; hybridization of 18S was included as a loading control. Quantification of TERRA signals normalized by 18S is shown in the bottom panel. The means and standard error of the means (s.e.m.) from independent experiments are indicated (n=number of independent experiments). The Student'st-test was used for statistical comparison (**P<0.01). C, control siRNA. (c) TERRA half-life after silencing hnRNP F was measured by incubating cells with actinomycin D, extracting total RNA at the time periods shown, and measuring TERRA levels by dot-blot analysis. The data were normalized to 18S rRNA levels and represented as a percentage of the TERRA levels measured at time 0, before adding actinomycin D, using a semilogarithmic scale. The mean and standard error of the mean (s.e.m.) of the percentage from three independent experiments are represented. The half-lives (t1/2) were calculated as the time required for TERRA to decrease to 50% of its initial abundance (discontinuous horizontal line). Figure 3: TERRA-bound RBPs regulate TERRA levels. ( a ) At 2 days after siRNA transfection, primary MEFs were harvested for western blot analysis to monitor RBP expression; whole-cell extracts (20 μg) were used to detect hnRNP A1 (A1), HuR (H) and hnRNP D/AUF1 (D) and nuclear extracts (50 μg) to detect hnRNP A2B1 (A2), hnRNP F (F) and hnRNP M (M). Duplicates of each transfection are shown. β-Actin was used as loading control. Quantification of RBP protein levels (%) relative to control transfection (C) is indicated in the bottom of each panel. ( b ) Northern blotting using a 32 P-dCTP-labelled 1.6 kb telomeric probe; hybridization of 18S was included as a loading control. Quantification of TERRA signals normalized by 18S is shown in the bottom panel. The means and standard error of the means (s.e.m.) from independent experiments are indicated ( n =number of independent experiments). The Student's t -test was used for statistical comparison (** P <0.01). C, control siRNA. ( c ) TERRA half-life after silencing hnRNP F was measured by incubating cells with actinomycin D, extracting total RNA at the time periods shown, and measuring TERRA levels by dot-blot analysis. The data were normalized to 18S rRNA levels and represented as a percentage of the TERRA levels measured at time 0, before adding actinomycin D, using a semilogarithmic scale. The mean and standard error of the mean (s.e.m.) of the percentage from three independent experiments are represented. The half-lives (t 1/2 ) were calculated as the time required for TERRA to decrease to 50% of its initial abundance (discontinuous horizontal line). Full size image To ascertain whether TERRA-bound RBPs could regulate TERRA location to telomeres, we performed immunofluorescence staining using antibodies against the TRF1 telomeric protein followed by RNA-fluorescence in situ hybridization (RNA-FISH) to detect TERRA ( Fig. 4 ). Interestingly, downregulation of hnRNP M and D/AUF1, and to a lower extent, hnRNP F and A2B1, caused a significant increase in TERRA foci co-localizing with TRF1, suggesting that these hnRNPs can block the location of TERRA to telomeres ( Fig. 4 ). As both hnRNP M and D/AUF1 have been previously shown to bind to single-stranded DNA [11] , [20] , [30] , absence of these two hnRNPs from telomeres may activate a mechanism that recruits TERRA to telomeres, possibly to increase telomere protection (see Fig. 5 for decreased telomere damage foci in hnRNP M and D/AUF knockdowns). 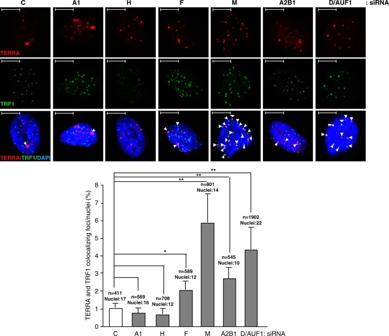Figure 4: Changes in TERRA location on TERRA-bound RBP downregulation. At 2 days after siRNA transfection, immunofluorescence followed by RNA-FISH was carried out to detect TERRA foci (red) and TRF1 protein (green). Arrowheads indicate co-localization events. The percentages of TERRA and TRF1 co-localizing foci per nuclei are represented (mean+s.e.m.). The total number of foci and nuclei used for the analysis are indicated. A total of three independent siRNA transfections were used for the analysis. The Student'st-test was used for statistical analysis (*P<0.05 and **P<0.01). The siRNAs used were: control (C), hnRNP A1 (A1), HuR (H), hnRNP F (F), hnRNP M (M), hnRNP A2B1 (A2B1) and hnRNP D/AUF1 (D/AUF1). Scale bars represent 5 μm. Figure 4: Changes in TERRA location on TERRA-bound RBP downregulation. At 2 days after siRNA transfection, immunofluorescence followed by RNA-FISH was carried out to detect TERRA foci (red) and TRF1 protein (green). Arrowheads indicate co-localization events. The percentages of TERRA and TRF1 co-localizing foci per nuclei are represented (mean+s.e.m.). The total number of foci and nuclei used for the analysis are indicated. A total of three independent siRNA transfections were used for the analysis. The Student's t -test was used for statistical analysis (* P <0.05 and ** P <0.01). The siRNAs used were: control (C), hnRNP A1 (A1), HuR (H), hnRNP F (F), hnRNP M (M), hnRNP A2B1 (A2B1) and hnRNP D/AUF1 (D/AUF1). Scale bars represent 5 μm. 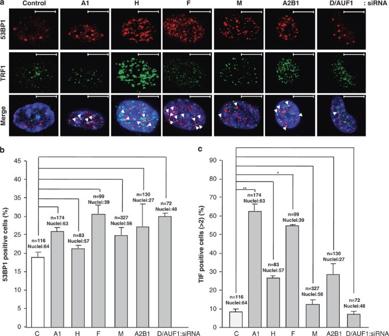Figure 5: TERRA-bound RBPs affect telomere capping. (a) Representative images of TRF1 (green) and 53BP1 (red) fluorescence, and of the merged images. Co-localization events (arrowheads), which represent telomere damage foci (TIF), are detected by yellow fluorescence. Scale bars represent 5 μm. (b) The mean and standard error of the mean (s.e.m.) of the percentage of 53BP1-positive cells and (c) percentage of more than two TIFs/nuclei are presented. Images are representative of graph fromFigure 5c. A total of three independent siRNA transfection experiments were used for the analysis. The Student'st-test was used for statistical analysis (*P<0.05 and **P<0.01). The siRNAs used were: control (C), hnRNP A1 (A1), HuR (H), hnRNP F (F), hnRNP M (M), hnRNP A2B1 (A2B1) and hnRNP D/AUF1 (D/AUF1). Full size image Figure 5: TERRA-bound RBPs affect telomere capping. ( a ) Representative images of TRF1 (green) and 53BP1 (red) fluorescence, and of the merged images. Co-localization events (arrowheads), which represent telomere damage foci (TIF), are detected by yellow fluorescence. Scale bars represent 5 μm. ( b ) The mean and standard error of the mean (s.e.m.) of the percentage of 53BP1-positive cells and ( c ) percentage of more than two TIFs/nuclei are presented. Images are representative of graph from Figure 5c . A total of three independent siRNA transfection experiments were used for the analysis. The Student's t -test was used for statistical analysis (* P <0.05 and ** P <0.01). The siRNAs used were: control (C), hnRNP A1 (A1), HuR (H), hnRNP F (F), hnRNP M (M), hnRNP A2B1 (A2B1) and hnRNP D/AUF1 (D/AUF1). Full size image Impact of TERRA-bound RBPs on telomere damage and length Next, we set out to assess the potential role of TERRA-bound hnRNPs in telomere protection by studying the presence of telomeric 53BP1 DNA damage foci (TIFs) after knockdown of the different RBPs. Although we did not detect significant differences in global DNA damage (see percentage of cells showing 53BP1 foci in Fig. 5a and b ), we detected a significant increase in telomere-co-localizing 53BP1 foci (TIF) on knocking down hnRNP A1, F and, to a lesser extent, when hnRNP A2B1 and HuR were targeted ( Fig. 5a and c ), indicative of increased telomere damage. Downregulation of hnRNP M and D/AUF1, however, did not lead to increased number of TIFs with respect to control cells. Interestingly, these two knockdowns were those that showed a more dramatic accumulation of TERRA to telomeres ( Fig. 4 ). These results suggest that the TERRA-bound RBPs may contribute to protect telomeres from eliciting a DNA damage response, and that to achieve this it is not sufficient to have increased TERRA levels or low mobilization to telomeres (as seen for hnRNP F siRNA; Figs 3b and 4 ), but a massive mobilization of TERRA to telomeres is also required (as in the case of hnRNP M and D siRNAs; Fig. 4 ). To ascertain whether changes in shelterin components contributed to the increased number of TIFs on downregulation of TERRA-interacting RBPs, we measured TRF1 and RAP1, two of the shelterin components, by immunofluorescence ( Supplementary Fig. S6 ). We did not observe significant changes in the co-localization of these two proteins except for an increase in the case of hnRNP M knockdown, in agreement with a higher TERRA localization to telomeres ( Fig. 4 ) and a very low abundance of TIFs in these cells ( Fig. 5a and c ). Finally, we also detected a decrease in RAP1/TRF1 co-localization events on hnRNP F knockdown, which may contribute to the high abundance of TIFs or uncapped telomeres present in these cells ( Fig. 5c ). Next, we addressed whether knockdown of the TERRA-interacting RBPs identified here resulted in altered telomere length. 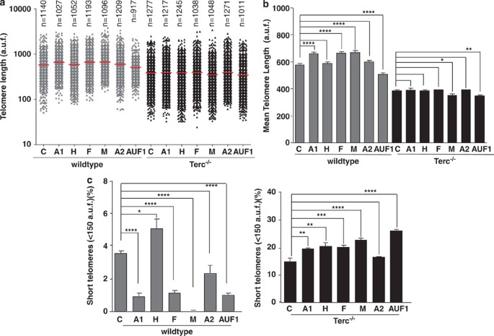Figure 6: TERRA-bound RBPs modify telomere length. (a) Telomere length calculated by quantitative FISH of individual telomere fluorescence distribution in interphase nuclei from the indicated siRNA-transfected primary MEFs. MEFs were obtained from wild-type andG1 Terc-null embryos33. The siRNAs used were: control (C), hnRNP A1 (A1), HuR (H), hnRNP F (F), hnRNP M (M), hnRNP A2B1 (A2B1) and hnRNP D/AUF1 (D/AUF1).n, number of telomeres used for the analysis for each RBP. Red bars, average telomere fluorescence intensity. a.u.f., arbitrary units of fluorescence. (b) Mean telomere length is also shown. (c) The mean and standard error of the mean (s.e.m.) of the percentage of short telomeres in wild-type (left) andG1 Terc−/−(right) siRNA-transfected primary MEFs. The number of telomeres (n) used inFigure 6b and cis shown inFigure 6a. The Student'st-test was used for statistical comparison of mean telomere length and theχ2-test was used to compare percentage of short telomeres (*P<0.05, **P<0.01, ***P<0.001 and ****P<0.0001). As shown in Figure 6a and b , knockdown of the different TERRA-interacting RBPs resulted in a significant increase in the average telomere length in the case of hnRNP A1, F, and M knockdowns. Furthermore, short telomeres were significantly decreased on downregulation of most TERRA-bound RBPs, except for HuR and hnRNP A2B1 (differences on hnRNP A2B1 knockdown did not reach significance) ( Fig. 6a and c ). These effects on telomere length were dependent on the telomerase status, as downregulation of TERRA-bound RBPs in first generation telomerase-deficient G1 Terc −/− MEFs [31] did not result in an increase in the average telomere length on hnRNP A1, F and M knockdowns and did not decrease the presence of short telomeres, as observed on similar knockdowns in wild-type littermates ( Fig. 6 ). Figure 6: TERRA-bound RBPs modify telomere length. ( a ) Telomere length calculated by quantitative FISH of individual telomere fluorescence distribution in interphase nuclei from the indicated siRNA-transfected primary MEFs. MEFs were obtained from wild-type and G1 Terc -null embryos [33] . The siRNAs used were: control (C), hnRNP A1 (A1), HuR (H), hnRNP F (F), hnRNP M (M), hnRNP A2B1 (A2B1) and hnRNP D/AUF1 (D/AUF1). n , number of telomeres used for the analysis for each RBP. Red bars, average telomere fluorescence intensity. a.u.f., arbitrary units of fluorescence. ( b ) Mean telomere length is also shown. ( c ) The mean and standard error of the mean (s.e.m.) of the percentage of short telomeres in wild-type (left) and G1 Terc −/− (right) siRNA-transfected primary MEFs. The number of telomeres ( n ) used in Figure 6b and c is shown in Figure 6a . The Student's t -test was used for statistical comparison of mean telomere length and the χ 2 -test was used to compare percentage of short telomeres (* P <0.05, ** P <0.01, *** P <0.001 and **** P <0.0001). Full size image Recent studies have revealed that non-coding RNAs containing UUAGGG repeats, named TERRA, are transcribed from telomeres that were largely thought to be transcriptionally inactive [5] , [6] . Several biological processes as well as cellular stresses have been described to influence TERRA levels and their nuclear localization and accumulation including the telomeric chromatin stage, telomere length, heat shock, exogenously inflicted DNA damage, as well as ontogenesis and cancer [6] , [8] , [32] (reviewed in Schoeftner and Blasco [9] ). However, the TERRA-bound factors controlling all of these processes remain largely unknown. A recent report described a number of proteins bound to TERRA in human cancer cells, including the telomere repeat-binding factor, TRF2, which was further shown to have a role in TERRA regulation. Here, we identify in primary MEFs a number of TERRA-interacting RBPs. In particular, we find that members of the hnRNPs, the ones that more abundantly bind to TERRA, influence TERRA levels by regulating the stability of the transcripts. Some of them also influence TERRA location at telomeres, which confers protection from telomeric DNA damage. Furthermore, knockdown experiments for each of the identified TERRA-bound RBPs also show a common role of hnRNPs on the telomerase-dependent elongation of short telomeres. While in preparation of this paper, a fraction of the TERRA-bound RBPs identified here in primary MEFs were also independently identified as TERRA-interacting proteins in human cancer cells, although they were not further studied by the authors [10] . These RBPs belong to the hnRNP family (hnRNP A1, A2/B1, M and U). The fact that members of the hnRNP family bind to both human and mouse TERRA suggest conservation among species and might be indicative of critical roles of hnRNPs in TERRA regulation. We show here that hnRNP A1, A2/B1, M and F are the proteins that bind more abundantly to TERRA, and they do so both in vitro and in vivo . The hnRNPs constitute a large family of proteins that were first found to be associated with nascent pre-mRNAs, packaging them into hnRNP particles. The hnRNPs particles were immunopurified by Dreyfuss' and co workers [30] in 1988 and are composed of an assortment of at least 24 polypeptides designated as hnRNP A1 to hnRNP U. The structural diversity of these proteins accounts for a multitude of functions that involve interactions with DNA or, more commonly, RNA. Most of them, if not all, are indeed single-stranded nucleic acid-binding proteins (preferentially RNA) [30] although with different nucleotide preference (for example, hnRP A1 and A/B bind to UUAGGG sequences, whereas hnRNP F favours XGGGX sequences). These binding preferences are in agreement with the binding of, for instance, hnRNP A1, A2/B1 and F to TERRA transcripts, which are composed of UUAGGG repeats. The hnRNPs are multifunctional and have been implicated in a wide variety of processes such as transcription, RNA processing, translation and signal transduction events (reviewed in Carpenter et al . [19] ). These proteins have also been associated with telomere biology because of their direct binding to telomeres, their interaction with the telomerase and their effect on telomere lengthening. In particular, hnRNP A1, A2B1, A3, D and E can associate with the single-stranded telomeric repeats, although only hnRNP A1 has been shown to influence telomere length [11] , [12] , [13] (reviewed in Ford et al . [14] ). The hnRNP A1, D and C1/C2 are also able to interact with human telomerase [12] , [15] , [16] , [17] , [18] and hnRNP A1 and D can unwind G-quadruplexes [18] , [20] . The hnRNP interaction with TERRA transcripts and the effects on TERRA and telomeres that we described here further support a central role of hnRNPs in telomere biology. Thus, we found that hnRNPs regulate TERRA abundance and localization, as well as influence telomere length. A direct effect of the hnRNPs on this process might be envisioned, as these proteins interact directly with TERRA, telomeres and telomerase [10] , [11] , [12] , [13] , [15] , [16] , [17] , [18] and because of the rapid effects observed 2-days on knockdowns, for instance, on the elimination of short telomeres. However, because of the cellular abundance of hnRNPs and their pleiotropic roles, we also expect global cellular changes on hnRNP knockdowns and, therefore, we cannot exclude the contribution of secondary players on the observed effects on TERRA and telomeres. Loss-of-function experiments described here suggest individual, as well as common roles for each of the different hnRNPs in TERRA and telomere regulation. In particular, we found that hnRNP F acts as a repressor of TERRA levels, at least in part, through the destabilization of the telomeric transcripts, although other transcriptional and post-transcriptional mechanisms cannot be discarded [19] . A different role was observed for hnRNP M and D. These two RBPs seem to block the access of TERRA transcripts to telomeres, as their downregulation increases the number of TERRA foci at telomeres. As discussed below, the mobilization of TERRA to telomeres maybe needed to protect telomeres when they become uncapped. We also found an apparent rescue of cells with short telomeres on knocking down most of the TERRA-interacting RBPs, which was dependent on the presence of telomerase. Although we cannot rule out that downregulation of TERRA-interacting RBPs may lead to elimination of cells with the shortest telomeres because of global effects of the knockdowns, these results may also suggest that hnRNP may influence either telomerase activity or the accessibility of telomerase to telomeres. Interestingly, some of the hnRNPs have been described to interact with human telomerase [12] , [15] , [16] , [17] , [18] . In addition, the results described here suggest a protective role of TERRA when mobilized massively to telomeres. In particular, although downregulation of TERRA-bound RBPs resulted in a significant increase in telomere dysfunction-induced foci (TIFs), such as in the case of hnRNP A1 and F, probably because of telomere uncapping (hnRNP A1, A2/B1 and D are known to bind single-stranded telomeric repeats), downregulation of hnRNP M and D, which strongly increased the mobilization of TERRA to telomeres, significantly protected them from TIF induction. These results suggest a protective role of TERRA at telomeres, which is in agreement with recent results showing that TERRA downregulation leads to increased TIFs [10] . Together, the results presented here show that TERRA transcripts are bound by a complex set of proteins, being hnRNP A1, A2B1, F and M the most abundant ones. In the past, different observations led to propose a model in which hnRNPs act as a molecular bridge or a linker to recruit telomerase to telomeres [14] , [17] , [29] . In light of our new findings that hnRNPs bind to TERRA transcripts, thereby affecting both their levels and their location, we would like to suggest additional levels of regulation to this model in which hnRNPs have distinct and common roles in TERRA stability, telomere protection and telomere length regulation. Cell culture and siRNA transfections The MEFs were obtained from wild-type embryos and G1 Terc -null embryos [33] at embryonic day E13.5, as previously described [31] . The target sequence for siRNA was 5′-AAGAGGCAATTACCAGTTTCA-3′ for HuR, 5′-ATGGATCAGAAAGAACATAAA-3′ for AUF1, 5′-CCACTTAACTGTGAAAAAGAT-3′ for hnRNP A1, 5′-AAGCTTTGAAACCACAGAAGA-3′ for hnRNP A2B1, 5′-AAACTTGTTACCTTCCATTAA-3′ for hnRNP F, 5′-ATGGAAGATGCTAAAGGACAA-3′ for hnRNP M and 5′-AATTCTCCGAACGTGTCACGT-3′ for control (C) siRNA; siRNAs (1.5 μg, Qiagen) were nucleofected with Amaxa system (Lonza), according to manufacturers' protocol, and cells were harvested 2 days later. Protein identification by MS Two MS approaches were used for identification of RBPs after pull-down assay: LC-MALDI-MS/MS analysis of pull-down material and MALDI TOF/TOF-MS analysis of excised bands obtained after SDS–PAGE separation and Comassie staining of pull-down material. A biotinylated control RNA corresponding to a random sequence of the same length (N48) as the biotinylated TERRA was used for differential identification. For protein identification from pull-down material, beads from six replicated assays were pooled and washed twice with ice-cold 25 mM ammonium bicarbonate. Bound proteins were chemically reduced by the addition of 20 μl of 10 mM DL -dithiothreitol at 65 °C for 1 h and alkylated by 50 mM iodoacetamide at room temperature in the dark for 30 min. Proteolytic digestion was then performed with 125 ng trypsin (Trypsin Gold, Promega) in 25 mM ammonium bicarbonate, with overnight incubation at 37 °C in a final volume of 50 μl. The reaction was stopped by adding 1 μl of 10% heptafluorobutyric acid. Digested samples were analyzed by LC-MALDI-MS/MS. Peptides were trapped into a 200 μm×5 mm monolithic capillary columns based on poly-(styrene/divinylbenzene) (PS-DVB) (PepSwift, LC-Packings) previously equilibrated in 0.065% heptafluorobutyric acid in water. Desalted peptides were separated on a 200 μm×50 mm PS-DVB column, using a lineal gradient from 100% buffer A (0.055% trifluoroacetic acid (TFA) in water) to 60% buffer B (0.055% TFA in 50% acetonitrile (v/v)) for 40 min at 2.5 μl min −1 at 60 °C. A total of 416 five-second fractions were spotted on a stainless steel plate together with 2.5 mg ml −1 α-cyano-4-hydroxycinnamic acid in 50% acetonitrile/0.1% TFA (v/v) and 5 mM ammonium dihydrogenphosphate, containing 10 fmol μl −1 Glu-fibrinopeptide (MW=1570.668 Da), as internal standard. Samples were subjected to MALDI MS/MS analysis using a 4800 Proteomics Analyzer equipped with TOF-TOF ion optics (Applied Biosystems/MDS Analytical Technologies) and 4000 Series Explorer V.3.5.1. The instrument was operated in positive ion reflector mode and calibrated with 25 fmol of Peptide Calibration Standard II mixture (Bruker Daltonik GmbH) and the above-mentioned Glu-fibrinopeptide as an internal standard. The laser power was set to 2,800 a.u. for MS and 3,600 a.u. for MS/MS with collision-induced dissociation on. MS spectra were acquired across the mass range of 700–3,600 Da, with a total accumulation of 2,000 laser shots and minimum S/N filter of 25 for precursor ion selection. MS/MS spectra were acquired for the 15 most abundant precursor ions, with a total accumulation of 4,000 laser shots for each precursor. For in-gel protein identification, proteins were isolated by SDS gel electrophoresis stained with Coomassie brilliant blue and processed as given in Shevchenko et al ., [34] and directly subjected to MALDI TOF/TOF-MS analysis. All MS/MS spectra generated were analyzed using ProteinPilot Software V2.01 rev 67476, with the Paragon search algorithm for interrogating the International Protein Index mouse database (release 20090225), using a detected protein threshold >2, expressed as unused ProtScore, (confidence >99%). Protein data sets were compared using ProteinCenter Software (Proxeon Bioinformatics A/S). Western blot analysis Whole-cell lysates and nuclear lysates were prepared using RIPA buffer and RSB buffer (10 mM Tris–HCl (pH 7.5), 10 mM NaCl, 3 mM MgCl 2 and inhibitors), respectively, as previously described [35] , [36] . Protein lysates were resolved by SDS–PAGE and transferred onto nitrocellulose membranes. Antibodies used were the following: hnRNP A1 (Sigma; 1:5000 dilution), HuR diluted in the ratio 1:1000 and hnRNP A2B1 diluted in the ratio 1:500 (Santa Cruz Biotechnology), hnRNP F diluted in the ratio 1:500 and hnRNP M clone 2A6 diluted in the ratio 1:1000 (Abcam), AUF1 (Upstate; 1:1000 dilution), and Vigilin (in-house; 1:1000 dilution). Following secondary antibody incubations, signals were visualized by enhanced chemiluminescence. IP assay of RNP complexes The IP assay was performed using nuclear extracts [37] , except that 100 million cells were used as starting material and the lysate supernatants were precleared for 30 min at 4 °C using 15 μg of IgG (Santa Cruz Biotechnology) and 50 μl of protein A-Sepharose beads (Sigma) that had been previously swollen in NT2 buffer (50 mM Tris (pH 7.4), 150 mM NaCl, 1 mM MgCl 2 and 0.05% Nonidet P-40) supplemented with 5% bovine serum albumin. Beads (100 μl) were incubated (18 h, 4 °C) with 30 μg of antibody and then for 1 h at 4 °C with 3 mg of cell lysate. After extensive washes with NT2 buffer and digestion of proteins in the IP material [38] , the RNA was extracted and used to perform northern blot. Antibodies used were the similar to those used for western blot analysis, except for hnRNP F that was from Santa Cruz Biotechnology (clone N15). Biotin pull-down analysis Biotin pull-down assays were carried out as described [39] by incubating 150 μg of nuclear lysate with 0.9 ng of biotinylated transcripts (Invitrogen) for 30 min at room temperature. A measure of 0.9 ng of total RNA was added as competitor. Complexes were isolated using streptavidin-conjugated Dynabeads (Dynal), and bound proteins in the pull-down material were analyzed either by MS or by western blotting. The biotinylated TERRA transcript consists of 8×UUAGGG; the control biotinylated transcripts consist of random RNA sequence not present in MEFs with the same length as that of TERRA transcript. See Western blot analysis section for antibodies used. Northern blot Total and nuclear RNA was isolated with Trizol or Trizol LS, respectively (Invitrogen) and northern blot analysis was performed using standard protocols. For detection of TERRA, random primer-labeled (Rediprime, GE Healthcare), a 1.6 Kb (TTAGGG) n cDNA insert excised from pNYH3 (kind gift from T. de Lange, Rockefeller University, NY), was used. Normalization of northern signals was performed with the 18S rRNA (Ambion). Northern signals quantification was carried out with ImageJ (NIH). mRNA stability Actinomycin D (5 μg ml −1 ) was added 2 days after siRNA transfection and total RNA was prepared at the time periods indicated; mRNA half-lives were calculated after quantifying dot-blot signals, normalizing to 18S rRNA levels, plotting on logarithmic scales and calculating the time period required for a given transcript to undergo a reduction to one-half of its initial abundance (at time zero, before adding actinomycin D). Immunofluorescence and immunostainings combined with RNA-FISH Cells grown on poly- L -lysine-coated coverslips (Becton Dickinson) were placed in cytobuffer (100 mM NaCl/300 mM sucrose/3 mM MgCl 2 /10 mM pipes (pH 6.8)) for 30 s, washed in cytobuffer with 0.5% Triton X-100 for 30 s, washed in cytobuffer for 30 s and then fixed for 10 min in 4% paraformaldehyde in phosphate-buffered saline (PBS). After washing with PBS, cells were blocked overnight at 4 °C in PBS containing 3% (w/v) bovine serum albumin, 0.1% Tween-20, 0.3 μg μl −1 tRNA (Invitrogen) and 0.8 μg ml −1 RNasin (Promega). Antibodies against mouse TRF1 (in-house, 1:500 dilution) were incubated in blocking solution for 60 min at 37 °C. The slides were washed twice in PBS Tween-20, overlaid with goat anti-rabbit IgG (Alexa 488; Invitrogen) diluted in the ratio 1:400 for 1 h in blocking solution at 37 °C, washed three times in PBS Tween-20 and post-fixed in 4% paraformaldehyde in PBS. The cells were dehydrated in 70, 80, 95 and 100% ethanol, air-dried and hybridized overnight at 37 °C with TERRA RNA probe in hybridization buffer (2× sodium saline citrate (SSC)/50% formamide). Slides were washed three times for 5 min in hybridization buffer at 39 °C, three times for 5 min in 2× SSC at 39 °C, 10 min in 1× SSC at 39 °C, 5 min in 4× SSC at room temperature, 5 min in 4× SSC containing 0.1% Tween-20 and DAPI (Molecular Probes) at room temperature and 5 min in 4× SSC at room temperature. Signals were visualized in a confocal ultraspectral microscope TCS-SP5 (Leica). RNA-FISH probe was generated by random priming (GE Healthcare) using the 1.6 Kb (TTAGGG) n cDNA (see 'Northern Blot') and Cy3-labelled dCTP (Amersham). When immunofluorescence only was carried out, the following antibodies were used: rabbit polyclonal 53BP1 antibody (Novus biological; 1:500 dilution), mouse monoclonal TRF1 antibody (Abcam; 1:200 dilution) and rabbit polyclonal RAP1 antibody (Bethyl; 1:200 dilution). Telomere length using telomere quantitative FISH on metaphases Telomere quantitative FISH on metaphases was performed as described [40] , [41] . The cutoff used in the determination of the percentage of short telomeres was determined by averaging the results obtained after subtracting the 25% percentile from the mean telomere length value in the different conditions. Polyadenylation assays A measure of 20 μg of total RNA was incubated with 60 pmol oligodT (Invitrogen) at 65 °C for 5 min followed by quick chill on ice for 5 min. Then, half of the sample was treated with 1 U of RNase H (Invitrogen) and the other half was left untreated. Both samples were incubated at 37 °C for 30 min and the digestion was stopped with EDTA. On RNA purification, changes in TERRA migration were detected by northern blot. How to cite this article: López de Silanes, I. et al . TERRA transcripts are bound by a complex array of RNA-binding proteins. Nat. Commun. 1:33 doi: 10.1038/ncomms1032 (2010).